Binary colloidal structures assembled through Ising interactions New methods for inducing microscopic particles to assemble into useful macroscopic structures could open pathways for fabricating complex materials that cannot be produced by lithographic methods. Here we demonstrate a colloidal assembly technique that uses two parameters to tune the assembly of over 20 different pre-programmed structures, including kagome, honeycomb and square lattices, as well as various chain and ring configurations. We programme the assembled structures by controlling the relative concentrations and interaction strengths between spherical magnetic and non-magnetic beads, which behave as paramagnetic or diamagnetic dipoles when immersed in a ferrofluid. A comparison of our experimental observations with potential energy calculations suggests that the lowest energy configuration within binary mixtures is determined entirely by the relative dipole strengths and their relative concentrations. The diverse functionality of crystalline materials found in nature has inspired the quest to develop man-made versions with building blocks ranging in size from atoms to bricks. The engineering of crystalline materials from nanometre to centimetre length scales, sometimes called metamaterials, have demonstrated unprecedented control over the propagation of light, sound and heat, making possible the construction of materials with novel macroscopic properties, such as photonic [1] , [2] , [3] , [4] or phononic [5] , [6] , [7] , [8] bandgaps (filtering), electromagnetic [9] , [10] , [11] and acoustic [12] , [13] , [14] cloaking (invisibility), and one-way propagation of optical [15] , [16] , [17] , acoustic [18] , [19] , [20] and thermal [21] , [22] , [23] energy (rectification). Despite the promise of this emerging class of materials, the methods for fabricating desired structures in a reliable and low-cost manner using nanometre or micrometre size building blocks remains a difficult challenge. Generally, the strategies for building artificial crystals are divided into two main classes: 'top-down,' which includes robotic assembly, lithography and moulding techniques; and 'bottom-up,' which relies on self-organization and directed assembly. Top-down techniques are well suited to building electromagnetic metamaterials that operate in the microwave regime [11] , [24] ; however, scaling these structures down to infrared and visible wavelengths has remained a significant challenge because the basic building blocks (or 'atoms') must be smaller than the operating wavelengths [25] , which brings both difficulty in patterning individual 'atoms' and a need to fabricate very large numbers of them to make a macroscopic device. Bottom-up colloidal self-assembly techniques present an attractive alternative to the top-down lithographic approaches for several reasons. First, colloids in the size range of 10 nm–10 μm can be fabricated through low-cost synthesis techniques and are of the appropriate length scale for achieving functionality at ultraviolet, visible and infrared wavelengths. Second, the pairwise interaction potentials of colloidal particles can be tuned to promote spontaneous assembly into a variety of two- and three-dimensional (3D) structures. Multi-component colloidal systems [26] , [27] , [28] , [29] , [30] , [31] , [32] , [33] , [34] , [35] (that is, 'colloidal alloys') as well as systems of particles with non-trivial internal structure, such as Janus particles [36] , [37] , [38] , [39] and particles with shape anisotropy [40] , [41] , [42] , are currently being explored due to their ability to tailor the particle interactions and enable the assembly of diverse crystalline structures. Current methods for assembling ordered structures with two or three particle types include kinetic techniques based on controlled drying [26] , [27] , [28] , [29] , [30] , [31] and thermodynamic techniques [32] , [33] , [34] , [35] , [43] , [44] that rely on spontaneous assembly into minimum free-energy configurations. Kinetic techniques using evaporation of a liquid meniscus have demonstrated a large variety of crystalline colloidal alloy structures [26] , [27] , [28] . However, the structural sensitivity to the evaporation rate, solvent type, surface tension and other parameters makes it challenging to reliably reproduce the desired structures. Free-energy minimization techniques, which involve tailoring the particle–particle interactions to spontaneously assemble into a desired crystal structure, have the potential for greater flexibility and reproducibility. The challenges there are to understand the necessary particle interactions, fabricate particles that manifest those interactions and develop techniques for avoiding metastable states in order to realize the equilibrium phase of interest. Ionic assembly techniques that are based on fixing the charges of two different particle types (one of each polarity) may offer the requisite programmability [32] , [33] ; however, these systems are difficult to anneal due to the narrow window for adjusting the temperature in aqueous fluids. In comparison with these previous techniques, electric and magnetic assembly techniques offer the unique ability to anneal dipolar colloidal assemblies by adjusting the external field strength, which has the effect of modulating the particle interactions and can induce melting of undesired metastable structures. Binary mixtures of polarizable spherical particles confined to a monolayer can spontaneously assemble into a variety of crystal structures, as reported in experiments [43] , [44] , [45] , [46] and simulations [47] , [48] . Previous work has focused primarily on centimeter-sized permanent magnets assembling at the air/liquid interface [45] , or on dielectrophoretic interactions between binary colloidal mixtures [43] . In the latter case, the frequency-dependent polarizability of the different particle types was used to adjust the antiferromagnetic interactions, causing like particles to repel and unlike particles to attract. However, only a few structures (honeycomb and square lattices, and one ring configuration) were experimentally observed. As an alternative, magnetic colloidal assembly systems have two key experimental advantages. First, the use of DC magnetic fields, as opposed to AC electric fields, allows for experiments to be conducted over long periods (hours) in isothermal, quasi-static conditions without fluid heating or other electro-hydrodynamic effects. Second, the ease of tuning the particle interactions in our magnetic colloidal assembly system by changing the fluid permeability and field strengths allows for exploration of a wider variety of thermodynamically favoured configurations than can be achieved with macroscale permanent magnets, which suffer from slow dynamics, limited control over the dipole moments and inability to adjust the interaction strength. Here, we analyze the process of crystal formation when a magnetic field is applied to a mixture of magnetic and non-magnetic spherical particles immersed in a ferrofluid, and we show that more than 20 different pre-programmed structures can be observed, including the kagome lattice, and several new chain states can be produced. Our experiments are largely explained by potential energy calculations using a model with just two parameters: the ferrofluid concentration and relative particle concentration. The good fit between theory and experiment suggests that the observed structures are energetically stabilized and that the assembly process can be effectively controlled. Preliminaries and notation The interaction energy within mixtures of monodisperse paramagnetic and diamagnetic spheres that are confined to a 2D monolayer is calculated assuming that all of the spins align in the direction normal to the layer. A necessary condition for forming large, single-domain crystalline structures is that the net dipole density in a unit cell of the crystal be close to zero. Meeting this condition avoids long-range repulsion between individual unit cells, allows the formation of larger crystals, and reduces the tendency to form polycrystalline mixtures of different phases. As a first-order approximation, we treat the particles as point dipoles confined to a single plane. When the dipole moments display out-of-plane orientations, the pairwise interaction energy is given by: which is an axially symmetric potential that bears some resemblance to ionic interactions, but with strengths that decay as r −3 . The dipole moments represent beads with either paramagnetic or diamagnetic properties, which depend on the bead properties relative to the surrounding ferrofluid. The moments of the beads are: where μ m , μ n and μ f are the absolute magnetic permeabilities of the paramagnetic bead (subscript m ), diamagnetic bead (subscript n ) and ferrofluid (subscript f ) in vacuum; H is the strength of an applied field, V is the volume of a particle and χ is the material's magnetic strength. In the system of interest, we have μ n ≈ μ 0 , the permeability of free space. Antiferromagnetic interactions, in which the unlike particles attract and the like particles repel, are produced when the following relationships are satisfied: μ m > μ f > μ n ≈ μ 0 , or in the short-hand notation when The potential energy of a unit cell in a crystalline configuration is determined from a Madelung summation: where superscripts a and r specify the attractive or repulsive interactions, respectively. Both the summation and the coefficients α mm , α nn and α mn depend on the particular lattice configuration. Previous works have adopted notation to classify convectively assembled binary colloidal systems, where LS, LS 2 and LS 13 (L and S refer to large and small spherical colloidal particles [33] ), for example, are the colloidal analogues of naturally occurring atomic structures, such as the NaCl, AlB 2 and NaZn 13 material systems. Here, we use the notation M x N y to indicate a lattice structure in which the unit cell contains x paramagnetic and y diamagnetic particles. The M x N y structures obtained by minimizing the total energy are consistent with our theoretical intuition that the potential energy can be minimized by maximizing the number of nearest neighbour contacts between dissimilar particles and minimizing the number of contacts between similar particles. Empirical investigations of binary colloidal assembly In our experiments, the two bead types are both ~1 μm in diameter. The paramagnetic bead consists of a polystyrene matrix impregnated with magnetic nanoparticles whereas the diamagnetic beads are pure polystyrene. The diamagnetic beads were slightly smaller than the paramagnetic beads though there was <10% difference in the size of the two bead types. The main difference is in their relative magnetic permeability with respect to the surrounding ferrofluid suspension. The magnetic permeability of the ferrofluid, μ f , was controlled by adjusting the volume fraction of suspended magnetic nanoparticles, φ f , which allows us to achieve the condition in which the paramagnetic and diamagnetic beads behave as 'up' and 'down' spins, respectively. We ignored other interactions such as gravity, as we conducted our experiments in thin fluid films of roughly 5 μm in thickness, which maintained the particles at approximately the same vertical position. We also ignored the van der Waals force because the structures melted when the external field was removed, indicating that magnetic interactions are dominant in this system. Fluid films were created by placing a 1.5-μl drop of bead mixture in between a glass slide and a cover slip. Mineral oil was placed around the edges of the fluid film in order to reduce fluid convection and evaporation, which allowed the assembly experiments to be carried out for several hours. Some example crystal structures that were observed experimentally are shown and illustrated in Fig. 1 . For better visualization of the assembled structures, we overlaid brightfield and fluorescence images. Only the non-magnetic beads contained a red fluorescent dye. For each crystal configuration, the net dipole density (dipole moment per unit area) is minimized when the ratio of the dipole magnitudes is inversely proportional to their relative concentrations within the crystal, ( n m / n n ). Example videos of binary crystals that have been produced are provided in Supplementary Movies S1 and S2 , which depict the assembly of MN square and MN 2 honeycomb tile phases, respectively, that form a few minutes after the application of a magnetic field. The tile structures were achieved by tuning the assembly conditions such that for the MN square tile phase, wherein the particles have equal moments and are integrated into the lattice in equal ratios, and for the MN 2 honeycomb tile phase, wherein the dipole moment of the magnetic bead is twice that of the non-magnetic bead, and they are incorporated into the lattice at a 1:2 ratio. Likewise, kagome lattices (MN 3 ) were formed for the experimental conditions: wherein the dipole moment of the magnetic beads is three times that of the non-magnetic beads, and they are incorporated into the lattice at a 1:3 ratio. 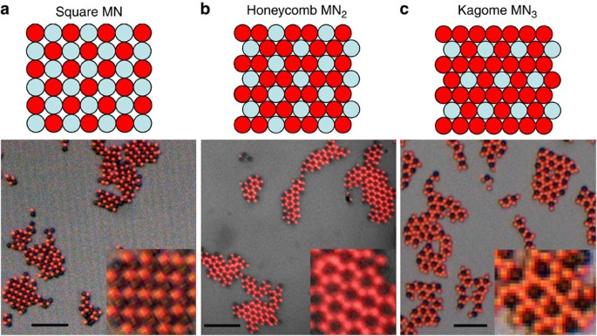Figure 1: Tile phases. Tile phases are observed when the relative dipole momentsare inversely proportional to the relative bead concentration,nm/nn. When the relative dipole moments are nearly equal, (a) square lattice (MN) is observed for the experimental conditions:in 3.5–4.5% volume fraction of ferrofluid. When the relative dipole moment of the magnetic bead is nearly twice that of the non-magnetic bead, (b) honeycomb lattice (MN2) is observed for the experimental conditions:in 1.7–2.3% volume fraction of ferrofluid. When the relative dipole moment of the magnetic bead is nearly three times that of the non-magnetic bead, (c) kagome lattice (MN3) is observed for the experimental conditions:in 1.2–1.3% volume fraction of ferrofluid. Illustrations of each lattice structure are provided, in which the magnetic beads are blue and the non-magnetic beads are red. Scale bar is 10 μm. Figure 1: Tile phases. Tile phases are observed when the relative dipole moments are inversely proportional to the relative bead concentration, n m / n n . When the relative dipole moments are nearly equal, ( a ) square lattice (MN) is observed for the experimental conditions: in 3.5–4.5% volume fraction of ferrofluid. When the relative dipole moment of the magnetic bead is nearly twice that of the non-magnetic bead, ( b ) honeycomb lattice (MN 2 ) is observed for the experimental conditions: in 1.7–2.3% volume fraction of ferrofluid. When the relative dipole moment of the magnetic bead is nearly three times that of the non-magnetic bead, ( c ) kagome lattice (MN 3 ) is observed for the experimental conditions: in 1.2–1.3% volume fraction of ferrofluid. Illustrations of each lattice structure are provided, in which the magnetic beads are blue and the non-magnetic beads are red. Scale bar is 10 μm. Full size image When the fluid cell was too thick, bilayers were sometimes observed, such as those shown in Fig. 2a . These multilayer structures indicate the tantalizing possibility of forming 3D ordered assemblies; however, image analysis in these systems is challenging due to the optical scattering of the ferrofluid, which interferes with diffraction techniques and confocal microscopy. Thus, in the majority of this work we restricted our attention to monolayer structures. When a horizontal field was applied to the suspension, a striped tile phase formed, consisting of alternating linear chains of magnetic and non-magnetic beads ( Fig. 2b ). 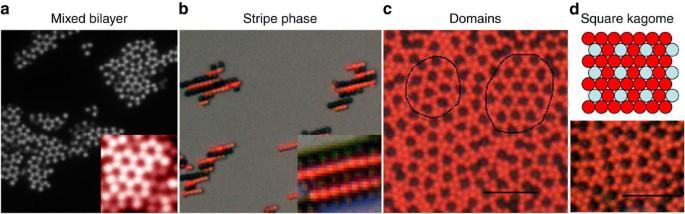Figure 2: Bilayers striped phases and kinetic assembly. When the fluid sample was too thick (a) bilayer structures formed, which can be visualized as the slightly brighter fluorescent spots that are produced by a stack of two fluorescent beads. A horizontally applied field of ~30 Oe produced (b) striped tile phase, consisting of alternating chains of magnetic and non-magnetic beads, which were observed for the experimental conditions:When the fluid was allowed to slowly dry, several non-equilibrium states could be observed, such as (c) a mixture of small domains of MN3kagome lattice surrounded by a colloidal glass, and (d) small domains of MN3-β square kagome lattice, which represents a higher-energy state than the more symmetric MN3kagome lattice structure. An illustration of the MN3-β structure is also provided. Scale bar is 10 μm. Striped chain phases were typically observed for the same conditions as the square lattice phase Figure 2: Bilayers striped phases and kinetic assembly. When the fluid sample was too thick ( a ) bilayer structures formed, which can be visualized as the slightly brighter fluorescent spots that are produced by a stack of two fluorescent beads. A horizontally applied field of ~30 Oe produced ( b ) striped tile phase, consisting of alternating chains of magnetic and non-magnetic beads, which were observed for the experimental conditions: When the fluid was allowed to slowly dry, several non-equilibrium states could be observed, such as ( c ) a mixture of small domains of MN 3 kagome lattice surrounded by a colloidal glass, and ( d ) small domains of MN 3 -β square kagome lattice, which represents a higher-energy state than the more symmetric MN 3 kagome lattice structure. An illustration of the MN 3 -β structure is also provided. Scale bar is 10 μm. Full size image When the net dipole density of the crystal diverges from zero, the dipole–dipole-induced strain between neighbouring unit cells causes the crystal to break up into multiple domains. This process is conceptually similar to electric and magnetic domain formation in solid state materials, such as antiferromagnetic and ferroelectric materials, where multiple domains can form as a result of a local excess of magnetization or electric polarization, respectively [49] . Mixtures of domains were sometimes observed for experimental conditions that are in between two lattice structures (that is, not completely optimized for a particular lattice configuration). For example, a mixture of MN 2 and MN 3 domains was observed for the experimental conditions: of 2 to 3. When the suspension was allowed to slowly dry, small crystalline domains surrounded by glassy regions were also observed, such as in Fig. 2c . Due to the kinetics of the drying process, we occasionally observed non-equilibrium states, such as the MN 3 -β square kagome tile structure ( Fig. 2d ), which has slightly higher-energy structure than the MN 3 kagome lattice as a result of the closer spacing of the magnetic beads. At even higher net dipole densities within a unit cell, a transition occurs in which chain phases become more energetical, because the density of contacts of unit cells within the chain phase is lesser compared with the tile phase. The types of chain phases that have been observed include MN 5 , MN 4 , MN 2 , MN and M 2 N structures ( Fig. 3 ). These structures represent chain variants of the kagome (MN 5 ), honeycomb (MN 4 , MN 2 and M 2 N) and square (MN) tile phases. Coexistence of chain and tile phases was observed in some of our experiments when the empirical conditions were in between the ideal conditions of nearby phases. Supplementary Movie S3 demonstrates the kinetics of the assembly process, in which the particles initially assemble in the MN 2 chain phase and then gradually rearrange into the MN 2 tile phase; however, coexistence of the MN 2 chain and tile phases was still observed even after long assembly times. 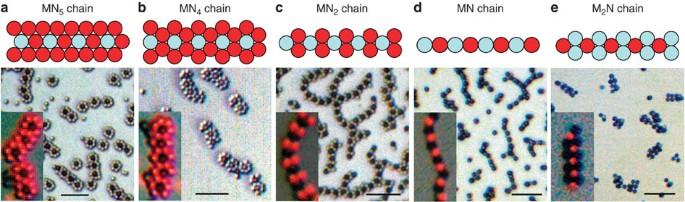Figure 3: Chain phases. Chain phases are observed when the relative dipole momentsare incompatible with the population ratio of 2D tile structures. When the relative dipole moment of the magnetic bead is nearly five times that of the non-magnetic bead, (a) kagome chain variant (MN5) is observed for the experimental conditions:in 0.9% volume fraction of ferrofluid. When the relative dipole moment of the magnetic bead is nearly four times that of the non-magnetic bead, (b) honeycomb chain variant (MN4) is observed for the experimental conditions:in 1.1% volume fraction of ferrofluid. MN2chain (c) is typically observed when the dipole moment of the magnetic bead is slightly larger than the non-magnetic bead and the concentration of the non-magnetic beads is slightly larger than the magnetic beads. This phase is often observed in coexistence with honeycomb and square tile phases for the experimental conditions:nn/nm≈1−2 andwhich occurs for 2.5–3.0% volume fraction of ferrofluid. MN chain phase (d) is observed rarely in experiments; however, one example is shown. When the dipole moment of the magnetic bead is roughly one half that of the non-magnetic bead, M2N chain phase (e) is observed, but often in coexistence with inverse honeycomb tile and/or square tile phase. The experimental conditions used to achieve the M2N chain structures wereat around 7% volume fraction of ferrofluid. Illustrations of each lattice structure are provided, in which the magnetic beads are blue and the non-magnetic beads are red. Scale bar is 10 μm. Figure 3: Chain phases. Chain phases are observed when the relative dipole moments are incompatible with the population ratio of 2D tile structures. When the relative dipole moment of the magnetic bead is nearly five times that of the non-magnetic bead, ( a ) kagome chain variant (MN 5 ) is observed for the experimental conditions: in 0.9% volume fraction of ferrofluid. When the relative dipole moment of the magnetic bead is nearly four times that of the non-magnetic bead, ( b ) honeycomb chain variant (MN 4 ) is observed for the experimental conditions: in 1.1% volume fraction of ferrofluid. MN 2 chain ( c ) is typically observed when the dipole moment of the magnetic bead is slightly larger than the non-magnetic bead and the concentration of the non-magnetic beads is slightly larger than the magnetic beads. This phase is often observed in coexistence with honeycomb and square tile phases for the experimental conditions: n n / n m ≈1−2 and which occurs for 2.5–3.0% volume fraction of ferrofluid. MN chain phase ( d ) is observed rarely in experiments; however, one example is shown. When the dipole moment of the magnetic bead is roughly one half that of the non-magnetic bead, M 2 N chain phase ( e ) is observed, but often in coexistence with inverse honeycomb tile and/or square tile phase. The experimental conditions used to achieve the M 2 N chain structures were at around 7% volume fraction of ferrofluid. Illustrations of each lattice structure are provided, in which the magnetic beads are blue and the non-magnetic beads are red. Scale bar is 10 μm. Full size image Both chain and tile phases become unstable at extreme dipole ratios (for example, ), in which case 0D ring configurations were predominantly observed. Some examples of ring structures are provided in Fig. 4 . Here, the packing fraction within the rings depended on n n / n m and in a manner consistent with past studies [44] . However, under some conditions the ring phases were also observed even at moderate dipole ratios. For example, R 4 ring structure was predicted theoretically and observed experimentally for the conditions and n n / n m ≈3. As another example, R 2 ring structure is predicted theoretically and observed experimentally near the conditions and n n / n m ≈1/7. 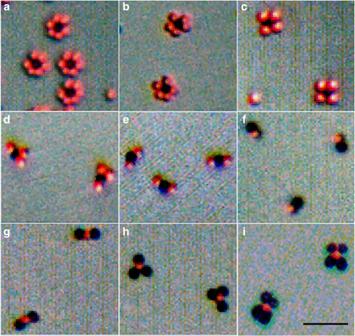Figure 4: Ring phases. The various ring phases that have been observed in experiments include: (a)R6, (b)R5, (c)R4, (d)R3, (e)R2, (f)R1, (g)R2*, (h)R3*and (i)R4*, where the subscript denotes the number of satellite particles in the ring and the * denotes an inverse ring configuration. Ring phases (a–f) were typically observed for large dipole moment ratios,(low ferrofluid concentrations <0.5%). The type of ring structures is controlled by varying the relative excess of non-magnetic beads. Inverse ring phases (g–i) were typically observed for small dipole m oment ratios(high ferrofluid concentrations >5%) and by controlling the excess of magnetic beads, such thatnn/nm<1. Scale bar is 5 μm. Figure 4: Ring phases. The various ring phases that have been observed in experiments include: ( a ) R 6 , ( b ) R 5 , ( c ) R 4 , ( d ) R 3 , ( e ) R 2 , ( f ) R 1 , ( g ) R 2 * , ( h ) R 3 * and ( i ) R 4 * , where the subscript denotes the number of satellite particles in the ring and the * denotes an inverse ring configuration. Ring phases ( a – f ) were typically observed for large dipole moment ratios, (low ferrofluid concentrations <0.5%). The type of ring structures is controlled by varying the relative excess of non-magnetic beads. Inverse ring phases ( g–i ) were typically observed for small dipole m oment ratios (high ferrofluid concentrations >5%) and by controlling the excess of magnetic beads, such that n n / n m <1. Scale bar is 5 μm. Full size image Theoretical phase diagram In order to explain these empirical results, we constructed a phase diagram based on the calculation of the potential energies of different structures as a function of the control parameters, and n n / n m . The results presented in Fig. 5 represent a T =0 phase diagram; entropic effects were not included. For each set of experimental conditions, we simulated the potential energy of more than 25 different structures that were chosen based on 2D close packing considerations (many of which were not observed in experiments), and the lowest-energy structure among these for each bead concentration and dipole moment ratio was used to produce the phase diagram. Nearest neighbour interactions were taken into account in computing the effective dipole moment of each particle in the unit cell (See Supplementary Tables S1–S3 ). The energy density of the lattice was calculated by summation of the pairwise interactions between all particles in an infinite crystal. Due to the fortuitous r −3 scaling of dipolar interaction energies, the energy density for a 2D system (with volume scaling as r −2 ) converged for sufficiently large lattice sizes (typically to within 1% for systems of 1,000 particles). 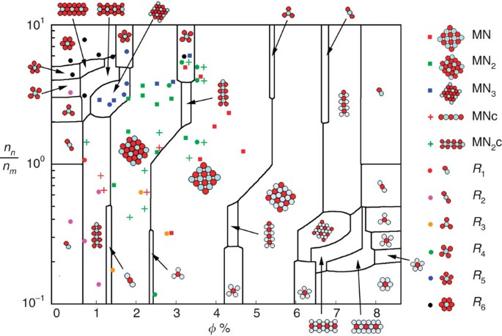Figure 5: Phase diagram. A computational phase diagram atT=0 predicts the stable regions of different tile, chain and ring phases. A description of the lattice energy calculations for each of the 25 simulated structures is provided in theSupplementary Methods.Supplementary Tables S1 through S3lists the effective dipole moments for each bead type that were calculated including nearest neighbour particle interactions for the tile, chain and ring phases, respectively.Supplementary Tables S4 through S6lists the energy densities for the tile, chain and ring lattice structures. The experimental data points (squares, crosses and circles represent tile phases, chain phases and ring phases, respectively) are overlaid on top of the theoretical phase diagram. The clustering of green squares, for example, shows the experimental conditions where honeycomb tile phase was predominantly observed (in 1.7–2.3% volume fraction of ferrofluid). The clustering of red squares shows the experimental conditions where square tile phase was predominantly observed (in 3.5–4.5% volume fraction of ferrofluid). Here,represents the ferrofluid volume fraction. We were unable to reliably explore the right-hand side of the phase diagram due to the requirement of large ferrofluid concentrations, which are several times in excess of the stock ferrofluid concentration (3.6% volume fraction); however, we provide theoretical predictions to show the type of structures that may be observed if different ferrofluids or particle types are used. Figure 5: Phase diagram. A computational phase diagram at T =0 predicts the stable regions of different tile, chain and ring phases. A description of the lattice energy calculations for each of the 25 simulated structures is provided in the Supplementary Methods . Supplementary Tables S1 through S3 lists the effective dipole moments for each bead type that were calculated including nearest neighbour particle interactions for the tile, chain and ring phases, respectively. Supplementary Tables S4 through S6 lists the energy densities for the tile, chain and ring lattice structures. The experimental data points (squares, crosses and circles represent tile phases, chain phases and ring phases, respectively) are overlaid on top of the theoretical phase diagram. The clustering of green squares, for example, shows the experimental conditions where honeycomb tile phase was predominantly observed ( in 1.7–2.3% volume fraction of ferrofluid). The clustering of red squares shows the experimental conditions where square tile phase was predominantly observed ( in 3.5–4.5% volume fraction of ferrofluid). Here, represents the ferrofluid volume fraction. We were unable to reliably explore the right-hand side of the phase diagram due to the requirement of large ferrofluid concentrations, which are several times in excess of the stock ferrofluid concentration (3.6% volume fraction); however, we provide theoretical predictions to show the type of structures that may be observed if different ferrofluids or particle types are used. Full size image For a given relative particle concentration, n n / n m , the excess particles of either type that could not be incorporated into a given lattice configuration were assumed to be infinitely far apart and thus produce a negligible contribution to the interaction energy. In our experiments, the free particles were typically found to remain several particle diameters away from the lattice, which makes this assumption plausible. More details on the calculation procedure along with a table of parameters for the energy density of each lattice type (tile, chain and ring, respectively) are provided in the Supplementary Tables S4–S6 . To convey the type of structures and the relative energies that we considered, Fig. 6 shows the potential energies as a function of the ferrofluid concentration. In this energy plot, the number ratio of non-magnetic to magnetic particles was taken to be n n / n m =1.5, and the external field was kept constant at 50 Oe. These calculations show that the system can adopt one of seven different lattice configurations as the ferrofluid concentration is increased. Near certain 'sweet spots' where a deep energy minimum for a particular phase is achieved, the difference in energy density between different lattice configurations was found to be substantial (as high as a few k B T ), which provides a qualitative explanation for why only one type of lattice structure was observed in certain experimental conditions. These energy calculations also show why coexistence of multiple different lattice configurations was observed near the certain phase boundaries: many structures have nearly the same energy in these regions. 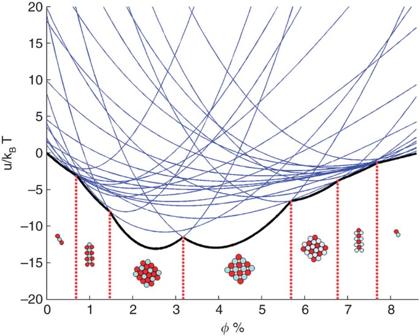Figure 6: Phase diagram potential energy diagram. The dimensionless potential energy of various structures is depicted for the particle ratio:nn/nm=1.5. The curves are calculated for an external field ofHext=50 Oe, temperatureT=298 K and particle sized=1 μm. The relatively deep potential energy minimum for several of the tile phases (square and honeycomb tile phases in particular) demonstrates why a single phase was predominant for many experimental conditions. The small potential energy difference near the boundaries indicates why coexistence of different phases was sometimes observed experimentally. Figure 6: Phase diagram potential energy diagram. The dimensionless potential energy of various structures is depicted for the particle ratio: n n / n m =1.5. The curves are calculated for an external field of H ext =50 Oe, temperature T =298 K and particle size d =1 μm. The relatively deep potential energy minimum for several of the tile phases (square and honeycomb tile phases in particular) demonstrates why a single phase was predominant for many experimental conditions. The small potential energy difference near the boundaries indicates why coexistence of different phases was sometimes observed experimentally. Full size image Figure 5 demonstrates that the potential energy calculations qualitatively account for the experimental data. The ferrofluid susceptibility was taken to vary linearly with the nanoparticle concentration, μ f = μ 0 (1+ φ f χ B ), where it was assumed that χ B =20 in accordance with specifications of the manufacturer and our previous work [44] , [50] . The magnetic permeabilities of the colloidal beads immersed in ferrofluid are more challenging to assess, as it is known that a thin magnetic nanoparticle coating can form on the bead surface (presumably due to a combination of hydrophobic and other surface interactions), which has the effect of modifying the magnetic permeabilities of the beads. While this effect may change the magnitude of interactions, the qualitative effect of reassigning the values of these two parameters ( μ n and μ m ) is just a horizontal stretching of the phase diagram. For convenience, in this work we simply assumed that μ m =2 μ 0 and μ n = μ 0 , which provided a reasonably good fit with experimental data. The actual particle ratio n n / n m was determined by counting the particles within each experimental image. There appears to be inversion symmetry within the phase diagram; however, the symmetry is not perfect due to the nonlinear scaling of the magnetic moments with the ferrofluid permeability, the nonlinearities being introduced by the denominator term in equation (2). Our calculations predict the correct experimental locations of the MN, MN 2 and MN 3 tile phases when the particle concentrations and dipole ratios were closest to the appropriate packing fractions, such as The ring phases are also in the correct locations for extreme ratios of for moderate ratios of the ring phases are also roughly in the correct place (particularly the R 4 and R 5 configurations). In other parts of the phase diagram, particularly near the boundaries of different phases, we frequently observed a coexistence of chain and tile phases, which could have resulted from a number of reasons. Experiments were typically performed near the effective melting temperature, based on theoretical insights obtained by others [48] . Theoretically, the lower field strengths should allow the structures to anneal more quickly by reducing energy barriers. However, the coexistence persisted in many experimental regions (particularly those in which the net dipole moment of a unit cell differed substantially from zero, that is, away from the 'sweet spots'), where the inclusion of entropic effects may be necessary for a more accurate calculation. The configurational entropy of meandering chain structures is expected to be larger than that of well-ordered crystals. A second possible experimental cause of the coexistence phenomena may have resulted from the relatively low bead concentrations used in experiments, as the average area fraction of particles in the monolayer regions was typically between 5–10%. Low particle concentrations were used in order to avoid particle stacking or the creation of bilayers, though these were sometimes observed due to slight density differences between the ferrofluid and the two particle types. In particular, the non-magnetic polystyrene particles presented a challenge as their density was close to that of the ferrofluid. We note that relatively low bead concentration encouraged the formation of small crystallites instead of a single large crystal or polycrystal. Liquid/solid phase transitions in most colloidal studies require a colloidal concentration close to 50%, thus the formation of small crystallites is not surprising in this case. It is also possible that the coexistence of the chain and tile phases in many regions of the phase diagram occurs only for low bead concentrations. The formation of small crystallites instead of one large crystal could also have resulted from the occasional defect in which particles adhering to the substrate acted as pinning sites for the nucleation of lattices or chains while at the same time limiting the growth of nearby structures. Particle–surface adhesion issues are an experimental artifact caused by the requirement of using extremely thin fluid films to offset the neutral density of the non-magnetic beads in ferrofluid. Future experimental enhancements could use thicker fluid films and denser non-magnetic particles (for example, silica or polymethyl methacrylate) that will allow both higher particle concentrations and reduce the incidence of particle adhesion issues that were introduced when the thin fluid samples were constructed. The main experimental challenge that limited our ability to fully explore the phase space of Fig. 5 was the high ferrofluid concentrations ( >6%) required to test the right-hand side of the phase diagram. We did observe other phases at the highest experimentally obtainable ferrofluid concentrations, including M 2 N and M 2 N-c tile and chain phases (see Fig. 3e ); however, the precise ferrofluid concentrations could not be reliably determined and the data are not included in the phase diagram. Despite these experimental and theoretical challenges, the key results we present are an empirical demonstration of the beginning of crystal formation in binary colloidal systems in which a diverse range of crystal structure can be produced by tuning two control parameters—relative particle moments and relative particle concentrations—and we developed a simple theory that explains the experimental observations. The sweet spots in the phase diagram where a clustering of tile phases were observed (green, blue and red squares) suggest that the experimental production of large single-domain crystals is possible. Although similar tile structures have been produced using alternative assembly techniques, such as the kagome lattice from surface-patterned Janus particles [36] , we present here the first examples of different kagome lattices assembled from bicomponent spherical isotropic particles. In addition, we observed a variety of chain and ring structures that have not been previously reported. The enhanced flexibility enabled by tunable Ising interactions within colloidal particle systems makes this work relevant not only to the exploration of fundamental problems in materials science and soft matter, but also to the bottom–up fabrication of photonic [26] , phononic [51] and magnetic [52] devices. Similar experiments using particles of different sizes may also open up a new realm of crystal structures that can be studied in quasi-equilibrium conditions, and provide fundamental insights into crystal formation in analogous materials at the atomic scale. Materials Magnetic beads (MyOne Dynal beads, Invitrogen) and non-magnetic beads (R100, Duke Scientific, Thermo Fischer), both having an approximate diameter of 1 μm, were supplied at concentrations of roughly 1% solids. In practice, the non-magnetic beads were about ~10% smaller than the magnetic beads, seen more clearly in the striped phase of Fig. 2b . We concentrated the beads by centrifugation and removed the effluent in order to achieve volume fractions of ~10%. The ferrofluid (EMG 707, Ferrotec, Nashua, NH, USA) is an aqueous magnetic nanoparticle suspension having a broad diameter distribution and a mean diameter of 12 nm [50] which was supplied at 3.6% volume fraction of solids. We were able to obtain concentrations of ferrofluid up to 12% solids by centrifuging the ferrofluid and removing the excess fluid; however, this led to increased ferrofluid aggregates and uncertainty over the final ferrofluid concentration. The beads and ferrofluid were mixed at different volumetric ratios; however, the total number of beads was kept constant in each experiment. For example, a relative particle concentration of n n / n m ≈1 in 1.8% volume fraction of ferrofluid was produced by mixing 5 μl of non-magnetic beads, 5 μl of magnetic beads and 10 μl of ferrofluid (see Table 1 ). We were principally concerned with the ratio of magnetic to non-magnetic beads, rather than the actual volume fraction of beads, and we did not attempt to confirm the actual volume fraction in the experiments, though it was in the neighbourhood of 5%. Negative volumes in Table 1 refer to the amount of water that was removed from the ferrofluid after centrifugation. The glass slides and cover slips were coated with a hydrophobic fluorocarbon that was deposited by vaporization of perfluorooctyltriethyoxylsilane (Alfa Aesar, Ward Hill, MA, USA) onto oxygen plasma cleaned glass slides, which served to reduce the adhesion of the colloidal beads to the fluid chamber walls. Table 1 Typical mixture ratios. Full size table Experimental apparatus Colloidal assembly experiments were observed in a 1.5-μl bead mixture placed between a glass slide and cover slip. To promote monolayer formation, the slide was gently pressed to create thinner fluid films. Mineral oil was placed around the edges of the fluid cell in order to prevent fluid convection and allow the experiments to be carried out for several hours in quasi-static conditions. Uniform magnetic field was applied to the fluid film by passing current through air-core solenoids (Fisher Scientific, Pittsburgh, PA, USA), which were mounted underneath the fluid cell. Microscopy was performed with a DM LM fluorescent microscope (LEICA, Bannockburn, IL, USA) using a ×40 air-immersion objective and a combination of brightfield and red filter cubes (Chroma Technology). The assembly process was conducted using fields of 30–70 Oe, which was kept close to the annealing field strength and thus is ideal for compact crystal growth. Larger fields led to frustration effects that prevented the formation of compact crystals. At the chosen fields, thermal agitation was sufficient to allow for particles to surmount metastable energy states and assemble into more thermodynamically favourable configurations. Data analysis The relative particle density ( n n / n m ) was determined using a Matlab code to count the magnetic and non-magnetic particles. Bright-field and fluorescent image files were imported as data files into a MATLAB program and a pixel-by-pixel analysis was used to identify the locations of each of the particles. A colour threshold was used to locate and count the beads, and the final output of the program was a bead count. The fluorescent images allowed for counting of the number of non-magnetic beads, whereas the bright-field images allowed us to count the number of magnetic beads. The tile, chain or ring structure that was predominantly observed in each image was designated as the most stable phase for that ferrofluid fraction and bead ratio. When multiple phases were present, each type of structure was recorded and the data were included in the phase diagram of Fig. 5 . The mixed phases are reflected in the grouping of nearby points, which we separated slightly so that the distinct phases could be graphically displayed. How to cite this article: Khalil, K. S. et al . Binary colloidal structures assembled through Ising interactions. Nat. Commun. 3:794 doi: 10.1038/ncomms1798 (2012).